Bottom-up formation of endohedral mono-metallofullerenes is directed by charge transfer An understanding of chemical formation mechanisms is essential to achieve effective yields and targeted products. One of the most challenging endeavors is synthesis of molecular nanocarbon. Endohedral metallofullerenes are of particular interest because of their unique properties that offer promise in a variety of applications. Nevertheless, the mechanism of formation from metal-doped graphite has largely eluded experimental study, because harsh synthetic methods are required to obtain them. Here we report bottom-up formation of mono-metallofullerenes under core synthesis conditions. Charge transfer is a principal factor that guides formation, discovered by study of metallofullerene formation with virtually all available elements of the periodic table. These results could enable production strategies that overcome long-standing problems that hinder current and future applications of metallofullerenes. Endohedral metallofullerenes (EMFs) exhibit properties that attract attention for use as contrast agents and other biomedical diagnostics, photovoltaics and materials [1] , [2] , [3] . EMFs are also of interest to the chemist, because the void within the cage acts as a nanoscale container for the study of remarkable structures and unusual systems [4] , [5] , [6] . Although first observed only days after the discovery of Buckminsterfullerene (C 60 ) [7] , [8] , the mechanism of metallofullerene formation remains unclear despite nearly three decades of intensive research, demonstrating the challenge of achieving in situ mechanistic insight under representative EMF-generating conditions. EMFs are synthesized in the gas phase from high-temperature, high-density carbon vapour by evaporation of metal-doped graphite [9] . All production methods involve creation of a carbon plasma with co-evaporated metal in the presence of an inert gas such as helium [7] , [10] , [11] . Therefore, the method of energy input used to vapourize graphite and metal is independent of the primary reactions that result in metallofullerene formation. It is generally established that a plasma serves as the starting point for synthesis by the electric arc discharge and laser vapourization techniques [7] , [10] , [12] . In fact, a distinct carbon–metal vapour (plasma) plume is physically observable during graphite evaporation [13] . Notably, one of the most vigorously exploited EMFs, M@C 82 (M=metal), has been macroscopically synthesized by the use of both methods since the dawn of metallofullerene science [12] , [14] . Top-down formation proposals have been predominantly advanced to explain fullerene synthesis over the past decade. By means of quantum chemical dynamics simulations, Irle et al . [15] concluded that spontaneous organization of giant carbon cages occurs first, after which C 2 elimination subsequently produces smaller fullerenes such as C 60 . Recently, Chuvilin et al . [16] demonstrated the transformation of graphene into a fullerene cage by electron beam irradiation in transmission electron microscopy studies. Very recently, Dorn and colleagues [17] isolated and characterized a metallofullerene proposed to be a key intermediate in the top-down formation of EMFs from graphite. However, we have recently reported that empty cages, such as C 60 and C 70 , may form through a different mechanism [18] . Here we present an alternate route to the formation of metallofullerenes, performed under characteristic synthesis conditions. We show that most known metal-encapsulated carbon cage sizes assemble through a bottom-up formation process. The prototypical M@C 82 metallofullerene is used to explicitly substantiate the nanocarbon reaction mechanism. More than 80 elements are individually investigated for mono-metallofullerene formation from metal-incorporated graphite to elucidate factors that control the process, in combination with density functional theory computations. Oxidation state of the encapsulated metal and charge transfer to the carbon cage are determinant factors that govern EMF formation. Molecular behaviour of Pr@C 82 in evaporated graphite vapour Pr@C 82 is synthesized by evaporation of Pr-doped graphite by the use of the electric arc plasma discharge technique. Two metal-encapsulated carbon cages are isolated from the resulting soot by chemical separation [19] , and then isomerically purified by multistep high-performance liquid chromatography (HPLC). The recovered species Pr@C 82 (I) and Pr@C 82 (II) [20] , labelled based on HPLC elution order, exhibit cages C 2v (9)-C 82 and C s (6)-C 82 . The Pr@C 82 compounds are described by an ionic model, in which valence electrons from Pr are formally donated to the cage, to give the charge distribution Pr 3+ @C 82 3− . These particular EMF cages are related by a single C 2 loss to the prominent M@C 80 cage (M=metal or cluster) [4] , [21] , [22] , [23] and are linked to all smaller endohedral fullerene cage sizes by further C 2 eliminations. By contrast, a single C 2 insertion reaction distinguishes Pr@C 82 from the larger M@C 84 cage [24] , [25] , [26] , and by further C 2 gain is connected to larger endohedrals [27] , [28] . Pr@C 82 occupies an intermediate position between well-known larger and smaller EMFs and provides an ideal platform to study the mechanism of metallofullerene formation. Mono-metallofullerenes offer compelling experimental evidence, because there is no ambiguity in product cage size [29] , [30] and the extent of charge transfer from metal to cage is well defined. 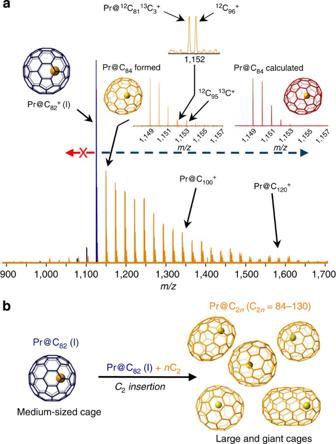Figure 1: Bottom-up formation of large and giant mono-EMFs from Pr@C2v-C82. (a) FT-ICR mass spectrum of cluster cations after reaction of Pr@C82with carbon evaporated from graphite in a low-pressure He atmosphere and (b) reaction scheme, with possible structures of the larger EMFs. The starting material is shown in blue, whereas bottom-up formation products are shown in orange. Figure 1 shows molecular cage behaviour and reactivity of Pr@C 82 (I) under synthetic conditions that generate EMFs, namely at high temperature, in the presence of carbon evaporated from graphite, and at a low-pressure of He. Direct sampling of the chemical formation process is achieved by the use of a pulsed laser vapourization source [18] , [31] , analysed by high-resolution Fourier transform ion cyclotron resonance (FT-ICR) mass spectrometry [32] . Pr@C 82 is unambiguously shown to undergo C 2 insertion reactions to form Pr@C 84 in high abundance, whereas a reverse reaction by C 2 elimination to Pr@C 80 essentially does not occur. All observed product EMFs display excellent agreement with calculated isotope distributions (inset in Fig. 1 ). Further, the results are consistent with previous investigations of medium-sized empty cage fullerenes (C 60 , C 70 , C 76 , C 78 , C 84 ) and the endohedral, La 2 @C 80 (ref. 18 ), which all exhibit growth into larger species without generation of smaller fullerenes in graphite vapour. As shown in Fig. 1 , extensive C 2 insertion reactions form EMFs significantly larger than Pr@C 84 , including giant metallofullerenes (>M@C 100 ). The endohedral nature of the Pr@C 2 n (C 2 n ≥C 84 ) products is confirmed by dissociation of isolated formation products ( Supplementary Fig. 1 ). Carbon nanostructures smaller than Pr@C 82 are primarily empty cages that result from bottom-up growth of C 80 , along with low abundance Pr@C 80 and Pr@C 78 . The species C 80 , Pr@C 78 and Pr@C 80 are attributed to result from an unavoidable interaction of the vapourization laser and the Pr@C 82 starting material, as indicated by Supplementary Figs 2 and 3 . Small M@C 2 n (C 2 n ≤76) species, although abundantly generated by vapourization of graphite, are entirely absent in Fig. 1 . Further, we note that those small endohedrals have received little study, because they are generally not detectable by use of the common arc discharge technique, as shown in Supplementary Fig. 4 . The second isomer, Pr@C 82 (II), exhibits similar behaviour under EMF synthesis conditions. Moreover, we have confirmed bottom-up formation of medium-sized cages to larger EMFs with other elements encapsulated in M@C 82 , such as Y@C 82 and Yb@C 82 . Figure 1: Bottom-up formation of large and giant mono-EMFs from Pr@ C 2v -C 82 . ( a ) FT-ICR mass spectrum of cluster cations after reaction of Pr@C 82 with carbon evaporated from graphite in a low-pressure He atmosphere and ( b ) reaction scheme, with possible structures of the larger EMFs. The starting material is shown in blue, whereas bottom-up formation products are shown in orange. Full size image M@C 2 n formation from metal-doped graphite Consequently, smaller compounds mark the start of EMF production from metal-doped graphite. 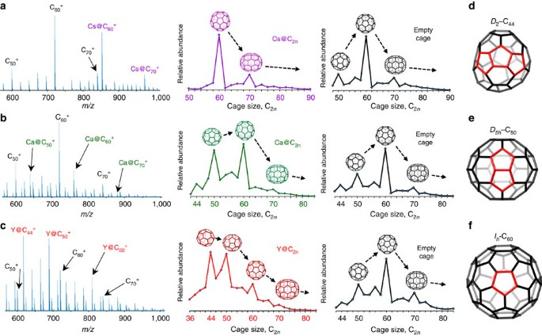Figure 2: Group 1–3 containing M@C2nfrom evaporated metal-doped graphite. Positive ions are representative of neutral distributions. M@C2nand C2ndistributions are shown graphically for each mass spectrum. As more negative charge is progressively transferred to the cage, as shown for (a) Cs+@C2n−, (b) Ca2+@C2n2−and (c) Y3+@C2n3−, non-IPR structures with particular pentagon motifs become highly stabilized and less reactive toward C2insertion. The proposed carbon cage for (d) M@C44contains four sets of TSFPs, (e) M@C50exhibits five sets of DFPs and all pentagons are isolated for (f) M@C60. Figure 2 shows fullerene synthesis products by laser evaporation of metal-incorporated graphite with representative elements from Groups 1, 2 and 3. All experiments are performed under similar formation conditions that result in a complex mixture of metallofullerenes and empty cages. EMFs that encapsulate a single metal atom ( Supplementary Fig. 5 ) range from M@C 28 to greater than M@C 100 in some cases, and all experimental distributions are highly reproducible (see Supplementary Fig. 6 ). The smallest M@C 2 n that form for a given element under the present conditions are shown in Figs 2 and 3 ; however, the largest M@C 2 n generally extend past ~M@C 84 . Experimental parameters are selected to yield C 60 as a dominant fullerene, thereby facilitating comparison of EMF with empty cage assembly and verifying consistent formation conditions among the large number of elements studied. In these strongly ionizing environments, positive ions are expected to be directly representative of neutral EMF distributions [7] . Supplementary Fig. 7 shows that calculated ionization potentials for Ca@C 2 n and Ti@C 2 n do not correspond to signal magnitude, providing additional support that observed M@C 2 n -positive ion distributions reflect neutral distributions. Figure 2: Group 1–3 containing M@C 2 n from evaporated metal-doped graphite. Positive ions are representative of neutral distributions. M@C 2 n and C 2 n distributions are shown graphically for each mass spectrum. As more negative charge is progressively transferred to the cage, as shown for ( a ) Cs + @C 2 n − , ( b ) Ca 2+ @C 2 n 2− and ( c ) Y 3+ @C 2 n 3− , non-IPR structures with particular pentagon motifs become highly stabilized and less reactive toward C 2 insertion. The proposed carbon cage for ( d ) M@C 44 contains four sets of TSFPs, ( e ) M@C 50 exhibits five sets of DFPs and all pentagons are isolated for ( f ) M@C 60 . 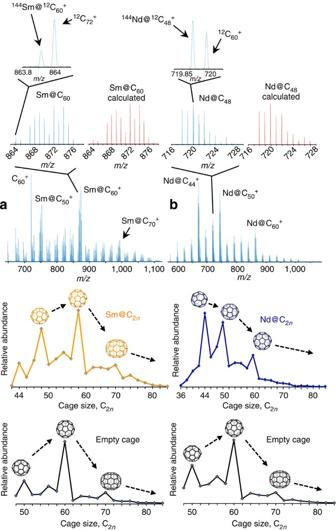Figure 3: Lanthanide-containing mono-EMFs from evaporated metal-doped graphite. Two distinct formation subsets are observed for lanthanides that involve transfer of two or three electrons to carbon cages, such as (a) Sm@C2nand (b) Nd@C2n. Full size image Figure 3: Lanthanide-containing mono-EMFs from evaporated metal-doped graphite. Two distinct formation subsets are observed for lanthanides that involve transfer of two or three electrons to carbon cages, such as ( a ) Sm@C 2 n and ( b ) Nd@C 2 n . Full size image Striking changes in formation distributions are observed for M@C 2 n across Groups 1, 2 and 3. Elements that formally donate a single electron to carbon cages, namely Na [33] , K, Rb and Cs ( Fig. 2a and Supplementary Figs 8–10 ) exhibit M@C 60 and M@C 70 as dominant species, similar to empty cages. By contrast, a considerable shift toward smaller EMFs occurs for elements that donate two electrons, as for Ca, Sr and Ba ( Fig. 2b and Supplementary Figs 11–13 ), in which M@C 50 becomes nearly as abundant as M@C 60 . Three-electron transfer to cages, as for Group 3 containing EMFs in Fig. 2c and Supplementary Figs 14 and 15 , affords a distribution that is more sharply skewed to smaller species, for example, highly abundant M@C 44 (for M=Sc, Y). All M@C 2 n synthesized from evaporated metal/graphite show outstanding agreement between calculated and experiment isotope distributions. M@C 82 is clearly observed for all elements that form endohedral fullerenes from graphite. Relative abundance of that compound can be enhanced by adjustment of formation conditions [18] , [34] (namely, by increasing laser fluence to create more available carbon vapour); however, small EMFs still dominate the products of formation. Therefore, the observed M@C 2 n trends are primarily equilibrium distributions under the present conditions, because most of the available carbon vapour formed should be able to react, that is, exhibit carbon insertion reactions with smaller M@C 2 n . It follows that there must be some point during the reaction that no ‘new’ small EMFs can be generated, but already formed M@C 2 n may still continue to grow bottom-up into larger species. Two distinct formation categories for the lanthanide series correspond to divalent and trivalent elements ( Supplementary Figs 16–29 ). Sm@C 2 n is representative of divalent lanthanide EMFs, M 2+ @C 2 n 2− . As shown in Fig. 3a , Sm@C 50 is formed in conspicuous abundance that rivals Sm@C 60 , a distribution pattern that mimics Group 2 EMFs. Nd@C 2 n , a representative element for trivalent lanthanide EMFs (Ln 3+ @C 2 n 3− ), is also shown in Fig. 3b . Nd@C 44 exhibits unusual abundance and an overall formation distribution that is nearly identical to Group 3 EMFs. We recently reported that Group 4 elements exhibit strongly altered formation distributions with the appearance of M@C 28 (ref. 35 ). Figure 3 demonstrates the ultra-high resolution of the present FT-ICR mass spectrometer that enables in situ investigation of many of these metal–carbon systems for the first time. Gas-phase isolation of M@C 2 n EMFs (C 2 n =44, 50, 60, 70, 80, 90) is carried out by the use of a stored waveform inverse Fourier transform event [36] . Subsequent structural investigation by sustained off-resonant irradiation collision-induced dissociation [37] confirms the endohedral location of elements inside the carbon cages ( Supplementary Note 1 ). Stored waveform inverse Fourier transform and sustained off-resonant irradiation collision-induced dissociation product ion mass spectra for M@C 60 with all EMF-forming elements are shown in Supplementary Figs 35–39 . Highly thermally excited M@C 60 does not produce the smaller unconventional ‘missing metallofullerenes’ M@C 28 , M@C 36 , M@C 44 or M@C 50 in significant abundance under our conditions, providing additional support for bottom-up formation of these species from graphite. Further support is gained through theoretical investigations probing bottom-up formation of the Ca@C 2 n family, as shown in Fig. 4 . 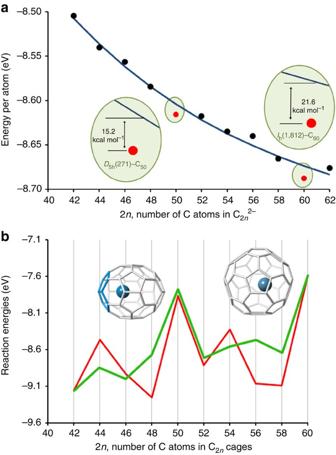Figure 4: Computational modelling of bottom-up formation for Ca@C2n. (a) Energy per atom for C2n2−dianions (2n=42–62) and (b) reaction energies for Ca@C2n+C2→Ca@C2n+2(2n=42–60). The computed values inaare fitted to an exponential function (blue line). The energies forD5h-C502−(271) andIh-C602−(1,812) isomers, shown as red dots, are found to be 15.2 and 21.6 kcal mol−1deviated from the general trend, indicating an enhanced stability. Inb, computed reaction energies (red line) are compared with experimental relative abundances (green line). Ca@D5h-C50(271) and Ca@Ih-C60(1812) are the least reactive species to C2insertion, in agreement with experimental observations. Figure 4: Computational modelling of bottom-up formation for Ca@C 2 n . ( a ) Energy per atom for C 2 n 2− dianions (2 n =42–62) and ( b ) reaction energies for Ca@C 2 n +C 2 →Ca@C 2 n +2 (2 n =42–60). The computed values in a are fitted to an exponential function (blue line). The energies for D 5 h -C 50 2− (271) and I h -C 60 2− (1,812) isomers, shown as red dots, are found to be 15.2 and 21.6 kcal mol −1 deviated from the general trend, indicating an enhanced stability. In b , computed reaction energies (red line) are compared with experimental relative abundances (green line). Ca@ D 5 h -C 50 (271) and Ca@ I h -C 60 (1812) are the least reactive species to C 2 insertion, in agreement with experimental observations. Full size image Figure 1 experimentally establishes transformation of medium-sized metallofullerene cages into large and giant species by C 2 insertion reactions, without formation of smaller EMFs. We propose that the smallest EMF compounds for a given element are the first to form by synthesis from evaporated metal-doped graphite. Ion mobility and other cluster source studies suggest that an evaporated metal ion nucleates carbon to initially form such small EMFs, in agreement with our observations [35] , [38] . Ensuing C 2 insertions into those small EMFs result in formation of medium-sized compounds, such as solvent-extractable M@C 82 , which is clearly the origin of large and giant EMFs formed through the bottom-up mechanism shown in Fig. 1 . Therefore, conversion of smaller EMFs into larger cages is crucial for synthesis of known endohedrals [39] , [40] . Figures 2 and 3 , and Supplementary Figs 8–33 show those important formation steps from evaporated graphite. Elements that form mono-metallofullerenes are displayed in Supplementary Fig. 5 and corresponding formation distributions are shown in Fig. 5 . We have recently reported Group 4 mono-metallofullerenes [35] . All Group 1–4 metals, lanthanides and actinides ( Supplementary Figs 30 and 31 ) form M@C 2 n from evaporated metal-doped graphite, except for Li, Be and Mg under the present conditions. We note, however, that a Li + @C 60 − material has been recently synthesized by Li + implantation into pre-existing C 60 (ref. 41 ). All other transition metals do not form EMFs from graphite in detectable abundance under the present conditions. Surprisingly, Ga and In are observed to encapsulate carbon cages ( Supplementary Figs 32 and 33 ). 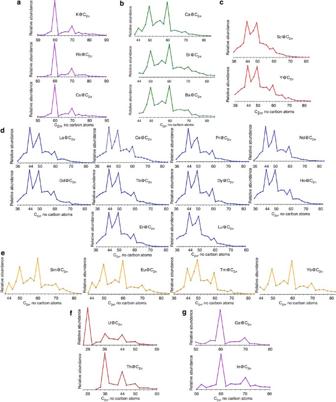Figure 5: M@C2nformation distributions with elements across the periodic table. Metallofullerene formation trends for (a) Group 1, (b) Group 2, (c) Group 3 metals, (d) trivalent lanthanides, (e) divalent lanthanides, (f) actinides, and (g) Ga and In from evaporated element-doped graphite. The smallest observed cages are shown for each M@C2n. The largest cages typically extend to ~M@C90or larger, but are not shown for simplicity. Figure 5: M@C 2 n formation distributions with elements across the periodic table. Metallofullerene formation trends for ( a ) Group 1, ( b ) Group 2, ( c ) Group 3 metals, ( d ) trivalent lanthanides, ( e ) divalent lanthanides, ( f ) actinides, and ( g ) Ga and In from evaporated element-doped graphite. The smallest observed cages are shown for each M@C 2 n . The largest cages typically extend to ~M@C 90 or larger, but are not shown for simplicity. Full size image Negative charge is preferentially located at pentagons or [5,6] bonds in the caged network of metallofullerenes, and to a greater extent when those pentagons are fused to result in [5,5] bonds and [5,5,5] junctions [42] . Consequently, charge transfer stabilizes highly pyramidalized C atoms induced by pentagon adjacency and cages that do not conform to the isolated pentagon rule (IPR) can become quite favourable systems [43] . All smaller fullerenes (<C 60 ) must possess various types of important fused pentagon motifs ( Fig. 2d–f ). Therefore, extent of charge transfer to double fused pentagons (DFPs), triple sequentially fused pentagons (TSFPs) and triple directly fused pentagons (TDFPs), and effect on C 2 insertion can be elucidated by in situ study of these small systems with various elements entrapped ( Figs 2 , 3 and 5 ). Particular significance is given toward tracking bottom-up transformation of M@C 28 →M@C 36 →M@C 44 →M@C 50 →M@C 60 by C 2 insertion reactions. The cage structure of T d -C 28 comprises exclusively TDFPs [35] , [44] , D 6 h -C 36 is the smallest cage that can exist without TDFPs [43] , [45] , D 2 -C 44 consists entirely of TSFPs motifs as described below, D 5 h -C 50 exhibits DFPs without TSFPs or TDFPs [46] , and I h -C 60 is the smallest in which all pentagons are isolated [47] . We have recently theoretically predicted that bottom-up construction of these smaller EMFs take place by exergonic C 2 insertions with free energy barriers that are attainable at the high temperature of synthesis [48] , providing strong support for the bottom-up mechanistic route. All possible isomers are computed for dianions, C 2 n 2− and Ca@C 2 n EMFs from C 42 to C 60 ( Fig. 4a and Supplementary Table 1 ), as recently done for tetravalent systems [48] , Ti@C 2 n . Carbon cages that encapsulate such divalent cations are advantageous for computational analysis because of the closed shell nature of their ground states. The computed values are fitted to an exponential function, as previously devised for hexanion EMFs [49] , to discern which Ca@C 2 n cages exhibit enhanced stability. We find that the relative energies of empty cage dianions and Ca@C 2 n follow the same trends and, therefore, the ionic model is applicable to Ca-encapsulated EMFs. Further, the most stable Ca@C 2 n and C 2 n 2− match the least-strained, lowest-energy empty cages; thus, although smaller EMF systems are described by charge transfer from the encapsulated metal to cage (for example, Ca 2+ @C 2n 2− ), strain is playing a major role in establishing the relative stability of isomers for a particular cage size. Many of the smaller EMF cages exhibit identical isomers to empty fullerene cages, permitting comparison of specific non-IPR isomer reaction paths [48] for EMFs with different metals encapsulated. Reaction energies for bottom-up, closed network growth [18] of Ca@C 2 n +C 2 →Ca@C 2 n +2 ( Fig. 4b ) show that specific isomers (also shown in Fig. 2d–f ) for Ca@C 50 and Ca@C 60 are the least reactive species to C 2 insertion, in agreement with experimental observations. In addition, we computed encapsulation energies ( Supplementary Table 2 ), which provide estimations of the interaction between the metal atom and carbon cage in EMFs, and determine that metal atoms with high oxidation states are favoured to encapsulate smaller cages. Encapsulation energies decrease when fewer electrons are formally donated to the cage and cannot compensate for the higher strain exhibited in small cages. Bottom-up growth of the medium-sized EMF, Pr@C 82 ( Fig. 1 ), exhibits considerably different reactivity towards C 2 insertions than do similar-size solvent-extractable empty cages, as known for C 84 and C 78 (ref. 18 ). The empty cages appear to grow much more rapidly than negatively charged cages (such as Pr 3+ @C 82 3− ). In essence, C 2 insertion becomes more difficult with increasing oxidation state of the encapsulated element and thus EMFs with carbon cages electronically described as C 2 n 3− ‘grow slower’ than empty fullerenes, in agreement with the changes in formation distributions with increasing negative charge on the cage for transformation of smaller M@C 2 n into medium-sized EMFs ( Figs 2 and 3 ) and theoretical modelling ( Fig. 4 ). Thus, charge transfer from metal to carbon cage and structural considerations can account for the fundamental M@C 2 n formation trends observed across the periodic table based on a bottom-up mechanism ( Fig. 5 ). Under synthesis conditions ( Figs 2 , 3 and 5 ) that give C 60 as the most abundant empty cage for C 2 n , medium-sized endohedrals, such as M@C 82 , are present in low relative abundance for mono-metallofullerenes, M@C 2 n . We interpret such ‘trapping’ of EMFs as non-extractable, smaller cages (for M@C 2 n , C 2 n <C 60 ) when sufficient charge is transferred by an encapsulated metal in the proposed bottom-up mechanism to be a major contributing factor to the low general yields of popular, solvent-extractable medium-sized and larger EMFs from evaporated graphite. On the other hand, that fundamental EMF formation property suggests that the abundant formation of smaller EMFs can be avoided by encapsulation of multiple elements or clusters of atoms, such as the M 3 N unit, to increase yield of solvent-extractable medium-sized or larger EMFs [4] . The metallofullerene formation ‘road map’ ( Fig. 5 and Supplementary Fig. 5 ) produced in this work should permit additional insight into the many unknown details of bottom-up EMF formation. For example, Ga and In are new elements discovered to incorporate in cages. Based on observed formation distributions, they are predicted to be uncommon Ga + and In + when encapsulated in carbon, as corroborated by DFT calculations ( Supplementary Fig. 34 ), and thus oxidation state of an encapsulated element may be identified by formation distributions. Such chemical information may be used to predict possible isomeric structures based on encapsulated metal. M III,IV @C 44 (M III,IV =trivalent or tetravalent metals) is found in unusual abundance when encapsulated by elements that donate three or more electrons to the cage ( Fig. 5 ). The prominence of C 28 , C 36 , C 50 , C 60 and C 70 resulting from evaporated graphite was essential for rationalizing the existence of empty cage fullerenes [47] . We interpret the emergence of the EMF C 44 cage ( Figs 2 , 3 , 4 , 5 ), to represent a previously unrecognized species that may be used to qualitatively understand the disparate behaviour of encapsulated metals in cages. The IPR rule was developed exclusively for pristine fullerenes but did not directly consider the TSFP motif ( Fig. 2d ) [47] . The unit of three sequentially fused pentagons is a linear triquinane that contains 11 carbon atoms [50] . Carbon cages require exactly 12 pentagons for closure and thus four sets of TSFPs bonded to each other would fulfill that fundamental constraint to yield a C 44 cage size. The resulting structure of C 44 , comprising exclusively TSFPs, should exhibit a special stability and would exist as a magic-numbered chemical system if properly stabilized, by analogy to cages D 5 h -C 70 , I h -C 60 , D 5 h -C 50 , D 6 h -C 36 and T d -C 28 , because neighbouring cage sizes (C 2 n ≤C 44 ) must contain more severely pyramidalized pentagon fusions. M@C 44 is the first EMF formed from smaller species in which all TSFP motifs are completely isolated from each other. The structure should be particularly stabilized to nucleophilic attack by C 2 and bond rearrangements in a bottom-up formation process when sufficient charge is acquired from an entrapped metal and plausibly explains the observed formation trends in Fig. 5 . Thus, the present results strongly suggest that M@C 44 exhibits cage isomer D 2 -C 44 (89) ( Fig. 2d ), which is predicted by DFT calculations [48] . Therefore, the linear triquinane (TSFP unit) should be found in other metallofullerenes, in addition to the known pentalene (DFP) motif [51] . Indeed, a particular recently isolated and characterized species of Sc 2 @C 66 displays two TSFP motifs [52] . The robust stabilization of various pentagon fusions in smaller metallofullerenes in the bottom-up formation scheme is in distinct contrast to empty cage formation and that mechanism can rationalize the structural origin of larger non-IPR EMF cages, as well as aid in prediction of EMF cage isomers for specific endohedral systems. Curious formation behaviour is observed for actinide-containing EMFs ( Fig. 5 and Supplementary Figs 30 and 31 ). Uranium is known to form the U@ T d -C 28 species, which is stabilized by transfer of four electrons to the cage [35] , [44] . Accordingly, it was predicted that thorium should exhibit similar behaviour, because its primary oxidation state is Th 4+ . Interestingly, Th@C 28 is not observed; however, Th@C 36 seems to have been essentially substituted ( Fig. 5 ) in the bottom-up formation path. This observation is likely due to the larger ionic radius of Th 4+ relative to U 4+ . The smallest cage that the Th 4+ ion can effectively nucleate must be greater than 28 carbon atoms, and in this case is Th@C 36 . The distribution of Th@C 2 n mimics U@C 2 n formation beyond Th@C 36 , which can now be explained by a similar extent of charge transfer during the bottom-up C 2 insertion process. M@C 28 is not observed for any rare earth encapsulated EMFs; however, Group 4 elements have been observed to encapsulate the C 28 cage [35] , in addition to U. Indeed, comparison of M@C 2 n with different groups is accurate in this respect, because, for example, very similar ionic radii exist for encapsulated elements such as Na + (1.02 Å), Ca 2+ (1.00 Å) and Ce 3+ (1.01 Å). Numerous other instances ( Fig. 5 ) of M@C 2 n with similar ionic radii but different oxidation states additionally support charge transfer as a determinant factor in bottom-up EMF formation. As shown in Fig. 5 , the smallest detectable cage(s) formed in abundance under the present conditions is M@C 50 for Group 1 elements (K, Rb, Cs), M@C 42 or M@C 44 for Group 2 elements (Ca, Sr, Ba), M@C 36 for trivalent rare earth metals (Sc, Y, La, Ce, Pr, Nd, Gd, Tb, Dy Ho, Er, Lu), although Sc@C 34 can be observed in very low abundance, M@C 44 or M@C 42 for divalent lanthanides (Sm, Eu, Yb, except Tm), and M@C 50 for Ga and In. These results also suggest that ionic radii may be a possible factor that alters EMF formation. In conclusion, we experimentally report that small, medium, and giant endohedral mono-metallofullerenes are formed in the gas phase from metal-doped graphite through a bottom-up mechanism under EMF synthesis conditions. The acquisition of negative charge from the encapsulated metal to cage, the hallmark of EMFs which give them spectacular properties, occurs at the inception of metallofullerene formation. Ionization energies of the elements appear to determine oxidation state after graphite/metal evaporation and thus extent of charge transferred to carbon cages, M n+ @C 2 n n− . Although strain energy is a trend-setting factor, particular smaller, unconventional EMFs become significantly stabilized by charge transfer, thereby impeding C 2 insertion reactions and thus inhibiting overall bottom-up formation of the small EMF compounds into solvent-extractable, larger metallofullerenes. The chemical manifestation also provides a natural explanation as to how non-IPR cage isomers may be formed for larger metallofullerenes. The understanding of EMF formation may bring into reality the ability to increase yield and drastically improve synthesis of particular molecular targets. There are still many unsolved aspects of metallofullerene formation that will require additional experimental evidence to elucidate, and further studies are underway in our laboratories. We note it is possible, and perhaps in some cases probable, that a C 2 loss event can occur in a bottom-up reaction path and thus should be necessary for a comprehensive explanation of fullerene formation. Molecular behaviour of M@C 82 in evaporated graphite M@C 82 (M=Pr and so on) was synthesized by the arc discharge technique. Pr@C 82 was isolated and purified by HPLC to yield the isomers Pr@C 82 (I) and Pr@C 82 (II). An isomerically purified sample of Pr@C 82 was then uniformly applied to the surface a pure graphite (99.9999%, 2–15 μm) target rod for carbon plasma exposure studies by use of an Nd:YAG laser (532 nm, 15 mJ per pulse) cluster source. Preparation and vapourization of metal-doped graphite Metal-incorporated graphite material (1–2 atomic % metal) is produced by combination of graphite (99.9999%, 2–15 μm) and, in most cases, metal oxide (≥99.9%). Metallofullerenes, M@C 2 n , are formed by evaporation of that metal-doped graphite material, after being moulded into a rod, by the use of an Nd:YAG laser (532 nm, 5 mj per pulse) in a pulsed cluster source. Cluster source and 9.4 T FT-ICR mass spectrometry Nanocarbon mechanism experiments are analysed with a custom-built FT-ICR mass spectrometer based on a 9.4-T superconducting magnet and performed with positive ions produced by a pulsed laser cluster source [18] , [33] , [35] . Evaporation of a translating and rotating target rod (12.7 mm diameter) is achieved by a single laser shot fired from an Nd:YAG (532 nm, 3–5 ns pulse width, ~1.5 mm beam diameter, 5–15 mj per pulse) in conjunction with the opening of a pulsed valve (800 μs duration) to admit He flow over the sample. Carbon vapour produced then enters a channel 4 mm in diameter and ~8.5 mm in length [18] . The laser is fired ~2 ms after opening of the pulsed valve for evaporation of metal-doped graphite samples and ~5 ms for M@C 82 -coated graphite samples. Ions accumulated by ten individual laser and helium pulse events are transported to an open cylindrical ion trap (70 mm diameter, 212 mm long, aspect ratio ~2). The ions are accelerated to a detectable cyclotron radius by a broadband frequency sweep excitation (260 Vp-p, 150 Hz μ −1 , 3.6 down to 0.071 MHz) and subsequently detected as the differential current induced between two opposed electrodes of the ICR cell. Each of the acquisitions is Hanning-apodized and zero-filled once before fast Fourier transform and magnitude calculation [53] . Ten time-domain acquisitions are averaged. The experimental event sequence is controlled by a modular ICR data acquisition system [54] . Ions are further probed by collision-induced dissociation. Computational details Amsterdam Density Functional code (ADF2011) was used [55] , [56] . The electronic density was provided by the local density approximation by use of Becke’s gradient-corrected exchange functional and Vosko–Wilk–Nusair parameterization for correlation, corrected with Perdew’s functional (BP86). Electrons for carbon and metals were described with Slater-type basis functions of triple-ζ polarization quality. We have included scalar relativistic corrections by means of the zeroth-order regular approximation formalism. How to cite this article: Dunk, P. W. et al . Bottom-up formation of endohedral mono-metallofullerenes is directed by charge transfer. Nat. Commun. 5:5844 doi: 10.1038/ncomms6844 (2014).